A smart and versatile theranostic nanomedicine platform based on nanoporphyrin Multifunctional nanoparticles with combined diagnostic and therapeutic functions show great promise towards personalized nanomedicine. However, attaining consistently high performance of these functions in vivo in one single nanoconstruct remains extremely challenging. Here we demonstrate the use of one single polymer to develop a smart ‘all-in-one’ nanoporphyrin platform that conveniently integrates a broad range of clinically relevant functions. Nanoporphyrins can be used as amplifiable multimodality nanoprobes for near-infrared fluorescence imaging (NIRFI), magnetic resonance imaging (MRI), positron emission tomography (PET) and dual modal PET-MRI. Nanoporphyrins greatly increase the imaging sensitivity for tumour detection through background suppression in blood, as well as preferential accumulation and signal amplification in tumours. Nanoporphyrins also function as multiphase nanotransducers that can efficiently convert light to heat inside tumours for photothermal therapy (PTT), and light to singlet oxygen for photodynamic therapy (PDT). Furthermore, nanoporphyrins act as programmable releasing nanocarriers for targeted delivery of drugs or therapeutic radio-metals into tumours. Nanoparticle-based theranostic agents are emerging as a promising paradigm towards personalized nanomedicine for disease- and patient-specific diagnosis and treatment [1] , [2] , [3] , [4] . The integration of imaging and therapeutic functions into a single nano-formulation allows precise diagnosis of disease, individualized selection of treatment modality, real-time monitoring of drug distribution/delivery and assessment of therapeutic outcomes [5] , [6] , [7] . Although conceptually impressive, these theranostic agents are still at an early stage of development. A variety of inorganic- and organic-based nanoparticles have been proposed; however, each type of nanoparticle displays distinct advantages and limitations. Inorganic nanoparticles often have unique physicochemical properties that allow applications in imaging and even therapy. For example, semiconductor quantum dots [8] , super paramagnetic iron oxide nanoparticles (SPIO-nanoparticles) [9] , [10] or gold-based nanomaterials [11] , [12] are valuable fluorescence probes, magnetic resonance imaging (MRI) contrast agents and photo-absorbers for photothermal therapy [11] , [12] , respectively. Although promising, these inorganic nanoparticles have not yet achieved broad clinical application because of concerns about their long-term safety and surface-dependent drug-loading property [7] , [13] . On the contrary, several ‘soft’ organic nanoparticles (for example, paclitaxel (PTX)-loaded polymeric micelles (Genexol-PM), liposomal doxorubicin (Doxil) and PTX-loaded human serum albumin nanoaggregate (Abraxane)) have been approved or are currently in clinical trials for the treatment of human cancers because of their excellent biocompatibility and drug-loading capacity. However, these organic nanoparticles have been used mainly as drug carriers since they generally lack imaging functions and intrinsic light absorbing ability for phototherapy. Additional efforts are usually needed to attach or encapsulate both therapeutic molecules and imaging agents [4] . Notably, a few organic nanoparticles, such as porphysome nanovesicles generated by porphyrin/lipid bilayers [7] and conductive polymer nanoparticles [14] , have recently been proposed as agents to transduce light to heat for photothermal therapy (PTT) against cancers. However, these nanoparticles tend to have high liver and spleen accumulation, in part because of their relatively large size (~100 nm), resulting in nonspecific clearance by the reticuloendothelial system, obviating the advantage of preferential tumour targeting over normal organs via enhanced permeability retention effect [15] , [16] , [17] . Furthermore, the theranostic nanoparticles reported thus far are only able to integrate limited number of clinically useful functions, thus narrowing their usefulness for diagnosis and treatment. Concerns also remain with many multifunctional nanoparticles regarding complexity of fabrication, unfavourable biodistribution and limited ability to regulate release of payload. In addition, high background noise and lack of an amplification strategy to increase the target’s signal output are major factors hampering advances in nanoparticle imaging functions [18] . There is a need for the development of biocompatible nanoplatforms that integrate a variety of recently advanced and clinically relevant imaging and therapeutic modalities. To successfully achieve multifunctionality, nanoparticles should be straightforward to prepare and ‘intelligent’ enough to overcome in vivo biological barriers such as interactions with blood proteins [19] , lipoproteins, blood cells, blood vessel walls and the reticuloendothelial system, and be able to deliver drugs and imaging agents efficiently in a targeted manner to diseased tissues. Here we report on a robust, smart and highly versatile ‘all-in-one’ porphyrin-based organic nanoconstruct (named nanoporphyrin, or NP) that can be constructed by using a single organic building block, a porphyrin/cholic acid (CA) hybrid polymer ( Fig. 1a,b ). This NP platform integrates a variety of imaging and therapeutic functions that include imaging (near-infrared fluorescent imaging (NIRFI), positron emission tomography (PET), magnetic resonance tomography (MRI), dual modal PET-MRI, PTT, photodynamic therapy (PDT), as well as targeted drug delivery ( Fig. 1a,b ). 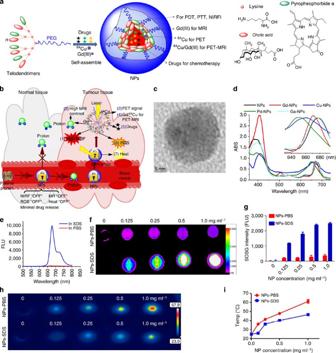Figure 1: Design, synthesis and characterizations of NPs. (a) Schematic illustration of a multifunctional NP self-assembled by a representative porphyrin–telodendrimer, PEG5k-Por4-CA4, composed of four pyropheophorbide-a molecules and four cholic acids attached to the terminal end of a linear PEG chain. (b) Schematic illustration of NPs as a smart ‘all-in-one’ nanomedicine platform against cancers. (c) TEM image of NPs (stained with phosphotungstic acid, PTA). (d) The absorbance spectra of NPs before and after chelating different metal ions. (e) Fluorescence emission spectra of NPs in the presence of PBS (red) and SDS (blue). Excitation: 405 nm. (f) Near-infrared fluorescence imaging of NP solution (10 μl) in the absence and in the presence of SDS with an excitation bandpass filter at 625/20 nm and an emission filter at 700/35 nm. (g) Single oxygen generation of NPs in PBS and SDS upon light irradiation (690 nm at 0.25 w cm−2for 60 s) measured by using SOSG as an indicator26,27(n=3). The results were expressed as the mean±s.d. Concentration-dependent photothermal transduction of NPs: (h) thermal images and (i) quantitative temperature change curve (n=2). The results were expressed as the mean±s.d. The temperature of NP solution (10 μl) in the absence and in the presence of SDS was monitored by a thermal camera after irradiation with NIR laser (690 nm) at 1.25 w cm−2for 20 s. Figure 1: Design, synthesis and characterizations of NPs. ( a ) Schematic illustration of a multifunctional NP self-assembled by a representative porphyrin–telodendrimer, PEG 5k -Por 4 -CA 4 , composed of four pyropheophorbide-a molecules and four cholic acids attached to the terminal end of a linear PEG chain. ( b ) Schematic illustration of NPs as a smart ‘all-in-one’ nanomedicine platform against cancers. ( c ) TEM image of NPs (stained with phosphotungstic acid, PTA). ( d ) The absorbance spectra of NPs before and after chelating different metal ions. ( e ) Fluorescence emission spectra of NPs in the presence of PBS (red) and SDS (blue). Excitation: 405 nm. ( f ) Near-infrared fluorescence imaging of NP solution (10 μl) in the absence and in the presence of SDS with an excitation bandpass filter at 625/20 nm and an emission filter at 700/35 nm. ( g ) Single oxygen generation of NPs in PBS and SDS upon light irradiation (690 nm at 0.25 w cm −2 for 60 s) measured by using SOSG as an indicator [26] , [27] ( n =3). The results were expressed as the mean±s.d. Concentration-dependent photothermal transduction of NPs: ( h ) thermal images and ( i ) quantitative temperature change curve ( n =2). The results were expressed as the mean±s.d. The temperature of NP solution (10 μl) in the absence and in the presence of SDS was monitored by a thermal camera after irradiation with NIR laser (690 nm) at 1.25 w cm −2 for 20 s. Full size image Synthesis and characterization of NPs NPs were formed by the self-assembly of a novel class of hybrid amphiphilic polymers (called telodendrimers) comprising linear polyethylene glycol (PEG) and dendritic oligomers of pyropheophorbide-a (Por, a porphyrin analogue) and CA ( Fig. 1a ; Supplementary Figs 1–3 ). PEG 5k -Por 4 -CA 4 , a representative telodendrimer, is shown in Fig. 1a and Supplementary Fig. 1 . Dynamic light scattering (DLS) showed the particle size of NPs to be ~21±6 nm ( Supplementary Fig. 4 ). On the basis of the molecular weight of telodendrimer and the total molecular weight of nanoparticle measured on DLS, we estimated that one NP nanoparticle was formed by the assembly of ~100 telodendrimers. Independently, transmission electron microscopy (TEM) showed that the NPs were spherical with a size of 21 nm ( Fig. 1c ) agreeing with DLS measurements. NPs have two absorption peaks, one at 405 nm and one in the near-infrared (NIR) range with peak at ~680 nm ( Fig. 1d ). PEG 5k -Por 4 -CA 4 has the intrinsic ability to chelate a variety of metal ions, such as copper (Cu(II)), palladium (Pd(II)), gadolinium (Gd(III)) and gallium (Ga(III)). Metal ion-loaded NPs, generated by the self-assembly of these metal-complexed telodendrimers in phosphate-buffered saline (PBS), were found to exhibit unique absorbance peaks ranging between 650 and 690 nm ( Fig. 1d ). When metal ions are loaded into the porphyrin components of the NPs, the heavy atoms show a higher scattering power, leading to more phase shift and higher contrast in TEM. Thus, the metal ion layer within the NP can be observed under TEM even without staining ( Supplementary Fig. 5 ). When excited at 405 nm, the NPs formulated in PBS showed a very weak red-fluorescence emission with a peak value at 680 nm ( Fig. 1e , red curve). This is not unexpected because of the π–π interactions and hydrophobic characteristics of Por molecules, which can easily form highly ordered structures in the interphase between the PEG corona and the hydrophobic core of the micellar NPs, contributing to the strong self-quenching effect of the excited state in the aqueous medium [20] . In contrast, when the NPs were disrupted by sodium dodecyl sulphate (SDS) [21] , [22] ( Supplementary Fig. 4 ), strong fluorescence at 680 nm was observed when excited at 405 nm ( Fig. 1e , blue curve). Figure 1f compares the NIR fluorescence of NPs as a function of NP concentration, with or without addition of SDS ( Supplementary Fig. 6 ). It is clear that NIR fluorescent signal of the NPs is greatly amplified upon micellar dissociation, which is expected to occur at tumour sites and/or inside the tumour cells. We have used our previously reported PEG 5k -CA 8 micelles [16] , [21] , [23] , [24] , [25] as a conventional micelle-based nanocarrier to physically encapsulate Por for comparison. NPs demonstrated 10 times more self-quenching than PEG 5k -CA 8 micelles (NM-POR) encapsulating the same concentration of Por ( Supplementary Figs 7 and 8 ), indicating quenching was a distinct characteristic of Por molecules that were assembled in the core of a NP construct. Similar to the fluorescence property, NPs also possess architecture-dependent ‘on/off’ photodynamic transduction. Generation of reactive oxygen species (ROS) by NPs in PBS after light irradiation was minimal but could be restored upon the addition of SDS, measured by using singlet oxygen sensor green (SOSG) as a highly selective singlet oxygen indicator ( Fig. 1g ) [26] , [27] . As NPs are highly self-quenched in PBS, energy is released in the form of heat instead of fluorescence and/or singlet oxygen generation upon laser irradiation ( Fig. 1h,i ). The temperature of the NP solution increased from 24 to 62 °C as NP concentrations increased from 0 to 1.0 mg ml −1 . When NPs were dissociated in the presence of SDS and illuminated with the same dose of light, strong fluorescence but less significant increase in solution temperature was observed ( Fig. 1h,i ). To the contrary, NM-POR only showed moderate temperature increase in PBS compared with that in SDS with the same level of illumination ( Supplementary Fig. 9 ), indicating that the photothermal transduction was efficient only when Por was confined to the interphase between the PEG corona and the hydrophobic core of the micellar NPs. Blood is the first biological barrier for nanoparticle-based drug delivery systems via intravenous administration. Interaction with blood proteins and lipoproteins may cause the dissociation of nanoparticles and lead to premature drug release [19] . In order to further increase the structural stability of NPs in blood circulation, we have applied reversible disulphide crosslinking strategy [19] , [21] to the NP platform. Four cysteines were introduced to the oligolysine backbone of the telodendrimer to form PEG 5k -Cys 4 -Por 4 -CA 4 ( Fig. 2a ; Supplementary Figs 10 and 11 ). The resulting NPs were then crosslinked via disulphide bond through oxidation of the thiol groups on the cysteines [21] , [28] . TEM showed that these disulphide-crosslinked NPs (CNPs) were spherical vesicles of 32±8 nm in diameter ( Fig. 2b ). Such CNPs retained their particle size even in the presence of SDS but were dissociated with the addition of both SDS and reducing agents ( Supplementary Fig. 12 ). Similar to the NPs, the fluorescence of CNPs was also highly quenched in PBS. Correspondingly, the fluorescence of CNPs was restored in the presence of both SDS and endogenous reducing agent such as glutathione (GSH) at intracellular levels [21] ( Fig. 2c ). 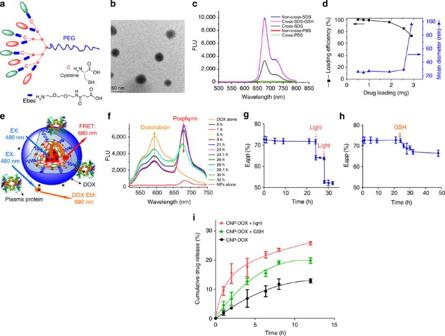Figure 2: Design, synthesis and characterizations of disulphide-crosslinked NPs. Schematic illustration of a representative crosslinkable porphyrin–telodendrimer (PEG5k-Cys4-Por4-CA4), composed of four cysteines, four pyropheophorbide-a molecules and four cholic acids attached to the terminal end of a linear PEG chain. Ebes was used as a spacer21. (b) TEM imaging of the disulphide-CNPs (stained with PTA). (c) The fluorescence emission spectra of the CNPs in the presence of PBS and SDS in the comparison with the non-CNPs. GSH was used as a reducing agent to break the disulphide crosslinking21. Excitation: 405 nm. These CNPs also showed very weak red-fluorescence emission with a peak value at 680 nm when excited at 405 nm (green curve). When the fluorescence emission spectra of the CNPs were recorded in the presence of SDS, there was increase in the peak emission at 680 nm (black curve). However, the peak value was significantly lower than that of the non-CNPs in the presence of SDS at the same porphyrin concentration. Upon addition of GSH, the CNPs were completely broken down and the peak at 680 nm in the fluorescence emission spectra increased further to a similar value as that of NPs in the presence of SDS (pink curve). (d) The loading efficiency of doxorubicin into CNPs and size change of doxorubicin-loaded CNPs (CNP-DOX) versus the level of drug-loading. The loading efficiency is defined as the ratio of drug loaded into nanoparticles to the initial drug content. The volume of the final NP solution was kept at 1 ml and the final concentration of the telodendrimer was 20 mg ml−1. (e) Schematic illustration of FRET-based approach for study of the real-time release of doxorubicin from nanoporphyrins in human plasma. FRET signal (f) and changes in apparent FRET efficiency (Eapp) (g) of CNP-DOX in human plasma with irradiation at 24 and 28 h, respectively (n=3). The results were expressed as the mean±s.d. Irradiation: 1.25 w cm−2for 5 min. The apparent FRET efficiency reflects the distance between the FRET pair and is calculated asEapp=IA/(IA+ID), whereIAandIDrepresent acceptor and donor intensities, respectively19. (h) Changes in apparent FRET efficiency (Eapp) of CNP-DOX in human plasma treated with GSH (10 mM) at 24 h (n=3). The results were expressed as the mean±s.d. (i) Cumulative DOX release profiles from CNP-DOX measured by dialysis method at 37 °C. Aliquots of CNP-DOX solution were pretreated with light (1.25 W cm−2, 5 min) or GSH (10 mM) or no treatment and then dialysed against diluted human plasma (n=3). The results were expressed as the mean±s.d. Data were reported as the average percentage of DOX accumulative release for each triplicate sample. Figure 2: Design, synthesis and characterizations of disulphide-crosslinked NPs. Schematic illustration of a representative crosslinkable porphyrin–telodendrimer (PEG 5k -Cys 4 -Por 4 -CA 4 ), composed of four cysteines, four pyropheophorbide-a molecules and four cholic acids attached to the terminal end of a linear PEG chain. Ebes was used as a spacer [21] . ( b ) TEM imaging of the disulphide-CNPs (stained with PTA). ( c ) The fluorescence emission spectra of the CNPs in the presence of PBS and SDS in the comparison with the non-CNPs. GSH was used as a reducing agent to break the disulphide crosslinking [21] . Excitation: 405 nm. These CNPs also showed very weak red-fluorescence emission with a peak value at 680 nm when excited at 405 nm (green curve). When the fluorescence emission spectra of the CNPs were recorded in the presence of SDS, there was increase in the peak emission at 680 nm (black curve). However, the peak value was significantly lower than that of the non-CNPs in the presence of SDS at the same porphyrin concentration. Upon addition of GSH, the CNPs were completely broken down and the peak at 680 nm in the fluorescence emission spectra increased further to a similar value as that of NPs in the presence of SDS (pink curve). ( d ) The loading efficiency of doxorubicin into CNPs and size change of doxorubicin-loaded CNPs (CNP-DOX) versus the level of drug-loading. The loading efficiency is defined as the ratio of drug loaded into nanoparticles to the initial drug content. The volume of the final NP solution was kept at 1 ml and the final concentration of the telodendrimer was 20 mg ml −1 . ( e ) Schematic illustration of FRET-based approach for study of the real-time release of doxorubicin from nanoporphyrins in human plasma. FRET signal ( f ) and changes in apparent FRET efficiency ( E app ) ( g ) of CNP-DOX in human plasma with irradiation at 24 and 28 h, respectively ( n =3). The results were expressed as the mean±s.d. Irradiation: 1.25 w cm −2 for 5 min. The apparent FRET efficiency reflects the distance between the FRET pair and is calculated as E app = I A /( I A + I D ), where I A and I D represent acceptor and donor intensities, respectively [19] . ( h ) Changes in apparent FRET efficiency ( E app ) of CNP-DOX in human plasma treated with GSH (10 mM) at 24 h ( n =3). The results were expressed as the mean±s.d. ( i ) Cumulative DOX release profiles from CNP-DOX measured by dialysis method at 37 °C. Aliquots of CNP-DOX solution were pretreated with light (1.25 W cm −2 , 5 min) or GSH (10 mM) or no treatment and then dialysed against diluted human plasma ( n =3). The results were expressed as the mean±s.d. Data were reported as the average percentage of DOX accumulative release for each triplicate sample. Full size image We have previously reported a series of CA-based telodendrimer nanocarriers for efficient encapsulation and delivery of anticancer drugs, such as PTX [21] , [23] , vincristine [25] and doxorubicin (DOX) [29] . We found that CNPs could also efficiently carry a variety of poorly water-soluble chemotherapeutic drugs and molecularly targeted drugs. For instance, DOX could be efficiently encapsulated inside CNPs with a loading capacity of 2.90 mg ml −1 ( Fig. 2d ). When formulated at 2.55 mg ml −1 , the drug-loading efficiency of DOX-loaded CNPs (CNP-DOX) was above 85% with final particle size ~30 nm ( Fig. 2d ). We then investigated the interaction of CNP-DOX with human plasma to simulate the destabilizing conditions in blood for in vivo applications and found that the particle size of CNP-DOX was highly stable ( Supplementary Fig. 13 ). We utilized the fluorescence resonance energy transfer (FRET) between the DOX and NPs to monitor the real-time drug release in human plasma ( Fig. 2e ). As shown in Fig. 2f,g , the FRET signal was very stable when CNP-DOX was incubated in human plasma for 24 h at 37 °C, indicating that the DOX release from CNPs was slow. However, there was dramatic and immediate FRET signal decrease with each light exposure at 24 and 28 h ( Fig. 2f,g ), indicating that CNPs could be triggered to release drug via illumination, probably as a result of local heat generation. As expected, DOX release could also be triggered by GSH at the intracellular level (~10 mM) [21] , as monitored with FRET ( Fig 2h ). We have also determined the release profiles of DOX from CNPs under similar conditions using the dialysis method [21] . Those results indicated that DOX release was slow in the presence of human plasma but could be facilitated through illumination or by adding GSH (~10 mM; Fig. 2i ). The DOX release profiles measured using the dialysis method were consistent with that determined with the FRET approach. Validation of NPs in cancer cell lines Intracellular delivery of CNP-DOX was investigated in SKOV3 ovarian cancer cells ( Fig. 3a ). After 2 h of incubation, DOX was released from CNPs and transported into the nucleus, while the NIR fluorescence from disassociated CNPs (unquenched telodendrimers) remained in the cytoplasm. To further study the relationship between the dissociation property of CNPs and intracellular GSH level, we conducted the cell uptake experiments on three cell lines: SKOV3 ovarian cancer cell line, PC3m prostate cancer cell line and MB49 mouse bladder cancer cell line. The order of GSH level of these cell lines is PC3m>SKOV3>MB49, as measured by an indicator, ThiolTracker Violet ( Supplementary Fig. 14 ). We found that in these cells intracellular GSH levels correlated positively with intracellular dissociation of CNPs, indicating that the disulphide crosslinks in CNPs are reversible. 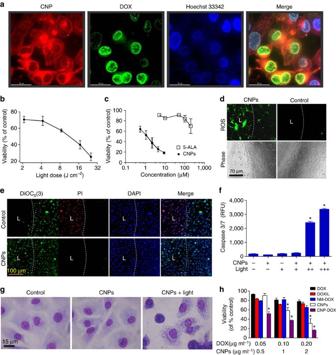Figure 3: Intracellular delivery and photocytotoxicity of NPs against cancer cells. (a) Uptake of DOX (green)-loaded CNPs (red) in SKOV3 ovarian cancer cell line. Cells were cultured in the eight-well chamber cover glass slides overnight. Cells were pretreated with Hoechst 33342 (blue) for 10 min for nucleus staining followed by incubation with CNP-DOX (DOX: 0.1 mg ml−1) in PBS. Imaging was acquired at 2 h using Deltavision deconvolution microscope (Scale bar=30 μm). The viability of SKOV3 ovarian cancer cells after (b) 2h exposure to 4.4 μM CNPs followed by illumination with various levels of NIR light, and (c) incubation with CNPs or 5-ALA for 24 h followed by exposure to NIR light at 0.07 W cm−2for 60 s. ROS-mediated cell death after CNPs and light treatment of SKOV3 ovarian cancer cells (n=3). The results were expressed as the mean±s.d. (d) Cells were treated with or without 2.2 μM CNPs for 24 h and loaded with DCF-DA for 30 min. After treatment with NIR light at 0.07 W cm−2for 60 s, images were acquired using fluorescence microscopy to detect ROS production; (e) SKOV3 ovarian cancer cells were incubated with 2.2 μM CNPs for 24 h in 96-well black-wall plate, stained with 40 nM of DiOC6(3) (Green, ΔΨmhigh) for 20 min at the end of incubation to evaluate mitochondrial membrane potential(ΔΨm), and followed by illumination of a portion of each well to elicit PDT effect. The illumination area was marked with ‘L’. Twenty-four hours later, the cells were stained with propidium iodide (PI) for cell death. (f) Cells were treated with different concentrations of CNPs for 24 h followed by PDT. Twenty-four hours later, caspase3/7 activity was measured by SensoLyte kit (Anaspec, Fremont, CA, USA) (n=3). The results were expressed as the mean±s.d. (g) Cell morphology after PDT. SKOV3 ovarian cancer cells were cultured on eight-well chamber slides and treated for 24 h with PBS, CNPs alone and combination of CNPs and light ( at 0.07 W cm−2for 60 s). Cells were then fixed and stained with Hema3 after 2 h. Cells treated with CNPs+light exhibited obvious nucleus swelling, cell rounding, membrane damage and cytoplasm aggregation. (h) Cytotoxicity effect from combination of doxorubicin with CNPs mediated phototherapy: SKOV3 ovarian cancer cells were treated with CNPs alone, CNP-DOX or doxorubicin-loaded standard micelles (NM-DOX)11with various concentrations of DOX and/or CNPs for 24 h. After washing, cells were exposed with light and cell viability was measured after 24 h (n=3). The results were expressed as the mean±s.d. *P<0.05, one-way analysis of variance (ANOVA). Figure 3: Intracellular delivery and photocytotoxicity of NPs against cancer cells. ( a ) Uptake of DOX (green)-loaded CNPs (red) in SKOV3 ovarian cancer cell line. Cells were cultured in the eight-well chamber cover glass slides overnight. Cells were pretreated with Hoechst 33342 (blue) for 10 min for nucleus staining followed by incubation with CNP-DOX (DOX: 0.1 mg ml −1 ) in PBS. Imaging was acquired at 2 h using Deltavision deconvolution microscope (Scale bar=30 μm). The viability of SKOV3 ovarian cancer cells after ( b ) 2h exposure to 4.4 μM CNPs followed by illumination with various levels of NIR light, and ( c ) incubation with CNPs or 5-ALA for 24 h followed by exposure to NIR light at 0.07 W cm −2 for 60 s. ROS-mediated cell death after CNPs and light treatment of SKOV3 ovarian cancer cells ( n =3). The results were expressed as the mean±s.d. ( d ) Cells were treated with or without 2.2 μM CNPs for 24 h and loaded with DCF-DA for 30 min. After treatment with NIR light at 0.07 W cm −2 for 60 s, images were acquired using fluorescence microscopy to detect ROS production; ( e ) SKOV3 ovarian cancer cells were incubated with 2.2 μM CNPs for 24 h in 96-well black-wall plate, stained with 40 nM of DiOC 6 (3) (Green, Δ Ψ m high ) for 20 min at the end of incubation to evaluate mitochondrial membrane potential(Δ Ψ m), and followed by illumination of a portion of each well to elicit PDT effect. The illumination area was marked with ‘L’. Twenty-four hours later, the cells were stained with propidium iodide (PI) for cell death. ( f ) Cells were treated with different concentrations of CNPs for 24 h followed by PDT. Twenty-four hours later, caspase3/7 activity was measured by SensoLyte kit (Anaspec, Fremont, CA, USA) ( n =3). The results were expressed as the mean±s.d. ( g ) Cell morphology after PDT. SKOV3 ovarian cancer cells were cultured on eight-well chamber slides and treated for 24 h with PBS, CNPs alone and combination of CNPs and light ( at 0.07 W cm −2 for 60 s). Cells were then fixed and stained with Hema3 after 2 h. Cells treated with CNPs+light exhibited obvious nucleus swelling, cell rounding, membrane damage and cytoplasm aggregation. ( h ) Cytotoxicity effect from combination of doxorubicin with CNPs mediated phototherapy: SKOV3 ovarian cancer cells were treated with CNPs alone, CNP-DOX or doxorubicin-loaded standard micelles (NM-DOX) [11] with various concentrations of DOX and/or CNPs for 24 h. After washing, cells were exposed with light and cell viability was measured after 24 h ( n =3). The results were expressed as the mean±s.d. * P <0.05, one-way analysis of variance (ANOVA). Full size image Without light irradiation, the intact CNPs showed no observable cytotoxicity up to 1.0 mg ml −1 against SKOV3 ovarian cancer cells, while free Por showed significant dark phototoxicity in a dose-dependent manner ( Supplementary Fig. 15 ). The efficacy of CNP-mediated PDT in vitro was found to be light-dose and CNP-dose-dependent ( Fig. 3b,c ). CNPs were much more cytotoxic than 5-aminolevulinic acid (5-ALA, an FDA-approved agent for PDT) using the same illumination dose ( Fig. 3c ). The loss of cell viability was found to be associated with intracellular ROS production ( Fig. 3d ), resulting in the loss of mitochondrial membrane potential, cellular damage and cell apoptosis as evidenced by caspase3/7 activation ( Fig. 3e–g ). Moreover, we found that CNP-DOX-mediated combination chemotherapy and phototherapy was significantly more efficacious than CNP-mediated phototherapy alone, free DOX or NM-DOX (DOX-loaded standard CA-telodendrimer-based micelles [21] without porphyrin) after illumination at corresponding doses of light ( Fig. 3h ). NP mediated multimodal imaging in animal models In order to exploit NPs as nanoprobes for in vivo imaging, it is important to first investigate their pharmacokinetics and biodistribution. In vivo blood elimination kinetic studies indicated that CNPs possess a longer circulation time in comparison with non-CNPs, indicating the enhanced in vivo stability of NPs with crosslinking ( Fig. 4a ). In order to quantitatively determine the distribution of NPs in tissues, Gd(III)-chelated non-crosslinked NPs (Gd-NPs) and Gd(III)-chelated CNPs (Gd-CNPs) were prepared and injected intravenously into nude mice bearing SKOV3 ovarian cancer xenograft. Twenty-four hours post injection, Gd concentration in tumour and normal organs was measured by inductively coupled plasma mass spectrometry. As shown in Fig. 4b , significant accumulation of Gd in the SKOV3 tumours was noted 24 h after Gd-NPs and Gd-CNPs administration in comparison with clinical formulation of gadolinium diethylenetriaminepentacetate complex (Gd-DTPA) designed for MRI imaging. Gd-CNPs accumulated 2.8 and 12.3 times more in tumour than Gd-NPs and Gd-DTPA, respectively. In addition, administration of Gd-CNPs resulted in significantly lower Gd uptake by the liver and spleen when compared with Gd-NPs and Gd-DTPA. Furthermore, it should be noted that in the Gd-CNPs group, Gd uptake by a tumour was much higher than that by the liver and the spleen. 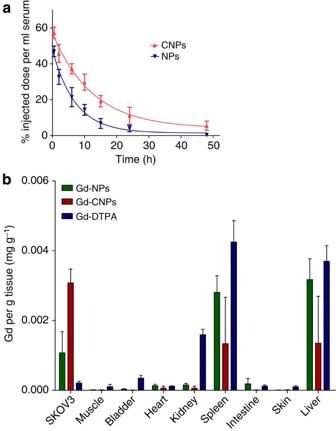Figure 4:In vivoblood elimination kinetics and biodistributions. (a)In vivoblood elimination kinetics of NPs and CNPs at a dose of 5 mg kg−1body weight (n=3 for each group). The results were expressed as the mean±s.d. (b) Gd distribution in tissues of SKOV3 ovarian cancer mice 24 h post injection of Gd-DTPA, Gd-NP and Gd-CNPs, measured by inductively coupled plasma mass spectrometry (ICP-MS, Agilent Techologies, 7500ce). Three mice were used in each experiment. Mice received Gd-DTPA, Gd-NP and Gd-CNP at the dose of Gd 20 mg kg−1. After 24 h, mice were killed. Tumour and major organs were collected and weighted. Tissue samples were treated with 200 μl of nitric acid under 60 °C for 2 h till most tissues were digested. Fat was digested by adding another 200 μl of 50% H2O2for 2–4 h and total volume was adjusted to 1 ml. Equal amounts of clear samples were used for ICP-MS analysis to detect Gd concentration. Results were normalized to original tissue weight and present as mg Gd per gram tissue (n=3 for each group). The results were expressed as the mean±s.d. Figure 4: In vivo blood elimination kinetics and biodistributions. ( a ) In vivo blood elimination kinetics of NPs and CNPs at a dose of 5 mg kg −1 body weight ( n =3 for each group). The results were expressed as the mean±s.d. ( b ) Gd distribution in tissues of SKOV3 ovarian cancer mice 24 h post injection of Gd-DTPA, Gd-NP and Gd-CNPs, measured by inductively coupled plasma mass spectrometry (ICP-MS, Agilent Techologies, 7500ce). Three mice were used in each experiment. Mice received Gd-DTPA, Gd-NP and Gd-CNP at the dose of Gd 20 mg kg −1 . After 24 h, mice were killed. Tumour and major organs were collected and weighted. Tissue samples were treated with 200 μl of nitric acid under 60 °C for 2 h till most tissues were digested. Fat was digested by adding another 200 μl of 50% H 2 O 2 for 2–4 h and total volume was adjusted to 1 ml. Equal amounts of clear samples were used for ICP-MS analysis to detect Gd concentration. Results were normalized to original tissue weight and present as mg Gd per gram tissue ( n =3 for each group). The results were expressed as the mean±s.d. Full size image The particle sizes of CNPs were ~32 nm ( Fig. 2b ), which is an optimal range for tumour targeting and penetration [15] , [16] . On the basis of their relatively small size, reversibly crosslinking nature and unique architecture-dependent fluorescence property, CNPs are particularly suitable to be used as activatable optical nanoprobes to increase the sensitivity of NIRFI for improved cancer detection through background suppression in blood, as well as preferential accumulation and signal amplification at the tumour site. The CNPs could stay silent (or in the OFF state) with minimum background fluorescence signals in blood circulation ( Fig. 5a , lower panel). The quenching status of CNPs in blood was further demonstrated by the recovery of fluorescence via the addition of SDS and GSH ( Supplementary Fig. 16 ). As expected, the overall fluorescence signal in the whole body was drastically lower for CNPs than non-CNPs after intravenous injection in nude mice bearing SKOV3 ovarian cancer xenograft ( Fig. 5a ). Upon accumulation at the tumour site via the size-mediated enhanced permeability retention effect, these crosslinked nanoprobes could be turned ON via the cleavage of disulphide bonds by the endogenous reducing agent GSH at the tumour site or in cancer cells [21] , followed by micellar dissociation and amplification of fluorescence signal ( Fig. 3a , Supplementary Fig. 14 ). CNPs showed significantly higher tumour accumulation than non-CNPs at 24 h post injection ( Fig. 5a ), in agreement with the biodistribution of Gd-loaded NPs ( Fig. 4b ). Ex vivo NIRF imaging at 24 h post injection showed that both non-CNPs and CNPs had superior fluorescence signal in tumours compared with normal organs ( Fig. 5b ). The average fluorescence signal of CNPs at the tumour site was 15.2 times higher than that in muscle of the same group of mice and 3.1 times higher than that of non-CNPs at the tumour site ( Fig. 5c ). The differential fluorescence signal between the CNPs and non-CNPs can be explained by the stability of the former construct in the circulation and higher uptake into the tumour ( Fig. 4a,b ). 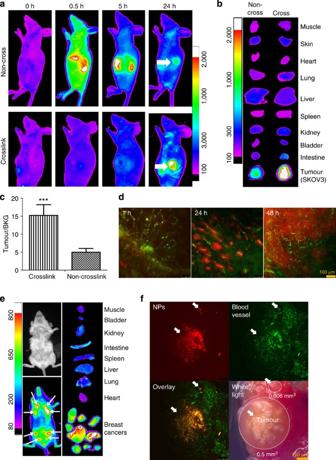Figure 5: Nanoporphyrin-mediated NIRF imaging in animal models. (a) Representativein vivoNIRF imaging of nude mice bearing SKOV3 ovarian cancer xenograft following intravenous injection of NPs and CNPs (NP dose: 25 mg kg−1). The white arrow points to the tumour site. (b) Representativeex vivoNIRF imaging of SKOV3 ovarian cancer xenograft 24 h post injection of NPs (left) and CNPs (right). (c) Quantitative NIRF fluorescence in tumour SKOV3 at 24 h post injection of NPs and CNPs (n=4; NP dose: 25 mg kg−1). Images were analysed as the average signal in the region of interest (ROI) in tumour and normalized to muscle. The results were expressed as the mean±s.d. ***P<0.001,t-test. (d) Projection images of the distribution of CNPs in SKOV3 tumour at 1, 24 and 48 h post injection observed by LSI laser scanning confocal microscope. Red: CNPs; Green: Dextran-FITC-labelled tumour blood vessel. (e) The representativein vivoandex vivoNIRF light imaging of transgenic mice with mammary cancer (FVB/n Tg(MMTV-PyVmT) at 24 h post injection of CNPs (NP dose: 25 mg kg−1). The white arrows point to the tumour site. Tumour volume was calculated by (L×W2)/2, whereLis the longest andWis the shortest tumour diameter (mm). (f) The accumulation of CNPs in lung metastasis of breast cancer in transgenic mice at 24 h post injection observed using LSI laser scanning confocal microscope. The white arrow points to the metastatic site. Red: nanoporphyrins; Green: Dextran-FITC-labelled tumour blood vessel. Figure 5: Nanoporphyrin-mediated NIRF imaging in animal models. ( a ) Representative in vivo NIRF imaging of nude mice bearing SKOV3 ovarian cancer xenograft following intravenous injection of NPs and CNPs (NP dose: 25 mg kg −1 ). The white arrow points to the tumour site. ( b ) Representative ex vivo NIRF imaging of SKOV3 ovarian cancer xenograft 24 h post injection of NPs (left) and CNPs (right). ( c ) Quantitative NIRF fluorescence in tumour SKOV3 at 24 h post injection of NPs and CNPs ( n =4; NP dose: 25 mg kg −1 ). Images were analysed as the average signal in the region of interest (ROI) in tumour and normalized to muscle. The results were expressed as the mean±s.d. *** P <0.001, t -test. ( d ) Projection images of the distribution of CNPs in SKOV3 tumour at 1, 24 and 48 h post injection observed by LSI laser scanning confocal microscope. Red: CNPs; Green: Dextran-FITC-labelled tumour blood vessel. ( e ) The representative in vivo and ex vivo NIRF light imaging of transgenic mice with mammary cancer (FVB/n Tg(MMTV-PyVmT) at 24 h post injection of CNPs (NP dose: 25 mg kg −1 ). The white arrows point to the tumour site. Tumour volume was calculated by ( L × W 2 )/2, where L is the longest and W is the shortest tumour diameter (mm). ( f ) The accumulation of CNPs in lung metastasis of breast cancer in transgenic mice at 24 h post injection observed using LSI laser scanning confocal microscope. The white arrow points to the metastatic site. Red: nanoporphyrins; Green: Dextran-FITC-labelled tumour blood vessel. Full size image Figure 5d shows projection images of the intratumoral distribution of the CNPs (red) obtained by large-scale-imaging (LSI) laser scanning confocal microscope. The tumour blood vessels were labelled with Dextran-FITC (green). The overall NIRF signal from CNPs was very low inside the tumour tissue at 1 h post injection ( Fig. 5d , left, Supplementary Movie 1 ). Significant NIRF signal was observed surrounding the blood vessels (green) at 24 h ( Fig. 5d , middle, Supplementary Movie 2 ), indicating the accumulation and partial dissociation of CNPs into tumour tissue around blood vessels. At 48 h, NIRF signals diffused throughout the entire tumour implying excellent tissue penetration and dissociation of CNPs at the tumour site ( Fig. 5d , right, Supplementary Movie 3 ). We further investigated the subcellular distributions of NPs in tumour tissue. The NIRF signal inside tumour cells was low at 24 h post injection of CNPs and increased significantly at 48 h post injection ( Supplementary Fig. 17 ). The fluorescence was mainly localized in the cytoplasm of cancer cells in a wispy to the focal pattern at 48 h post injection of CNPs. These results demonstrated the excellent delivery of NPs to target tumour cells after intravenous injection. We then investigated the NIRF-imaging capability of CNPs in transgenic mice (10–12 weeks) with naturally occurring breast cancers (FVB/n Tg(MMTV-PyVmT)) through intravenous injection. After 24 h, high fluorescence was observed in all the spontaneous breast cancers ( Fig. 5e ), as CNPs accumulated in the tumours and inside the tumour cells, they dissociated and became unquenched. Ex vivo imaging further confirmed the preferential uptake of the CNPs in all nine excised breast tumours compared with normal organs after 24 h. In some experiments, we used older transgenic mice (20–24 weeks) and detected accumulation of NPs in metastatic lesions in the lungs with LSI laser scanning confocal microscope, including tiny lesions that measured less than 100 μm in diameter ( Fig. 5f ; Supplementary Fig. 18 ). The NPs have intrinsic ability to chelate Gd(III) ( Fig. 1d ), preferentially accumulate at the tumour sites and possess architecture-dependent magnetic resonance properties that permit their use as activatable contrast agents for sensitive and tumour-specific MRI. Similar to the fluorescence measurements in Fig. 1e,f , there is low MRI signal enhancement when Gd-NPs retain their micellar integrity in PBS ( Fig. 6a ). This is likely because of the stacking of Gd/Por at the interface between the hydrophobic core and hydrophilic corona, thus shielding Gd(III) from interacting with protons in water. Upon dissociation in SDS, the Gd ion chelated by the Por has access to nearby protons and therefore shorten their spin-lattice relaxation time, resulting in an enhancement of the MRI signal ( Fig. 6a ). This unique architectural feature of Gd-NPs offers the opportunity for sensitive MRI detection of tumour as the background signal of the circulating NPs is low. We validated the application of Gd-NPs for MRI in transgenic mice with ‘spontaneous’ mammary cancers. A set of representative slices at different time point post injection is shown in Fig. 6b . We demonstrated that Gd-NPs could significantly enhance the contrast of tumour at 1.5 h post injection with very low signal enhancement in normal tissue. The tumour contrast was sustained for more than 26 h. Doses of Gd used in these studies were equivalent to 1/7th of the clinically recommended Gd dose for human [30] . These results confirm that the MRI signal enhancement in the whole body is low when the Gd-NPs are circulating in blood. After reaching the tumour site or tumour cells, the Gd-NPs dissociate and allow the interaction of Gd ions with surrounding protons, resulting in the significant MRI contrast only at the tumour site ( Fig. 1b ). The above data demonstrated that Gd-NPs even without crosslinking have excellent performance as contrast agents for tumour-specific MRI. Gd-CNPs are expected to have even better properties for MRI than Gd-NPs because of superior tumour accumulation ( Fig. 4b ). The investigation of Gd-CNPs as MRI contrast agents in animal models is on-going in our laboratory. 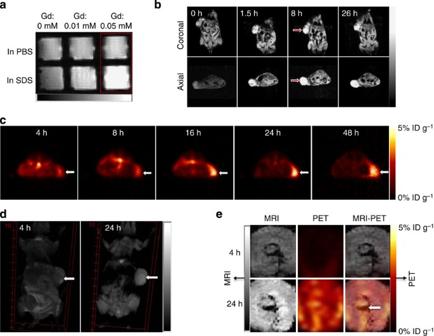Figure 6: Nanoporphyrin-mediated MRI and PET imaging in animal models. (a)In vitroMRI signal of Gd-NPs in the absence and in the presence of SDS obtained by T1-weighted MRI on a Bruker Biospec 7T MRI scanner using a FLASH sequence. (b) Representative coronal and axial MR images of transgenic mice with mammary cancer (FVB/n Tg(MMTV-PyVmT) using a FLASH sequence pre-injection and after injection of 0.15 ml Gd-NPs (Gd dose: 0.015 mmol kg−1). The white arrow points to the tumour site. (c) PET image of nude mice bearing SKOV3 ovarian cancer xenografts at 4, 8, 16, 24 and 48 h post injection of64Cu-labelled NPs (150–200 μl,64Cu dose: 0.6–0.8 mCi). The white arrow points to the tumour site. (d) 3D coronal MR images of nude mice bearing A549 lung cancer xenografts using a FLASH sequence at 4 or 24 h post injection with 0.15 ml of64Cu and Gd dual-labelled NPs (150–200 μl,64Cu dose: 0.6–0.8 mCi, Gd dose: 0.015 mmol kg−1). The white arrow points to the tumour site. (e) PET-MR images of tumour slices of nude mice bearing A549 lung cancer xenograft at 4 or 24 h post injection of dual-labelled NPs. White arrow points to the necrotic area in the centre of the tumour. Figure 6: Nanoporphyrin-mediated MRI and PET imaging in animal models. ( a ) In vitro MRI signal of Gd-NPs in the absence and in the presence of SDS obtained by T1-weighted MRI on a Bruker Biospec 7T MRI scanner using a FLASH sequence. ( b ) Representative coronal and axial MR images of transgenic mice with mammary cancer (FVB/n Tg(MMTV-PyVmT) using a FLASH sequence pre-injection and after injection of 0.15 ml Gd-NPs (Gd dose: 0.015 mmol kg −1 ). The white arrow points to the tumour site. ( c ) PET image of nude mice bearing SKOV3 ovarian cancer xenografts at 4, 8, 16, 24 and 48 h post injection of 64 Cu-labelled NPs (150–200 μl, 64 Cu dose: 0.6–0.8 mCi). The white arrow points to the tumour site. ( d ) 3D coronal MR images of nude mice bearing A549 lung cancer xenografts using a FLASH sequence at 4 or 24 h post injection with 0.15 ml of 64 Cu and Gd dual-labelled NPs (150–200 μl, 64 Cu dose: 0.6–0.8 mCi, Gd dose: 0.015 mmol kg −1 ). The white arrow points to the tumour site. ( e ) PET-MR images of tumour slices of nude mice bearing A549 lung cancer xenograft at 4 or 24 h post injection of dual-labelled NPs. White arrow points to the necrotic area in the centre of the tumour. Full size image Furthermore, NPs have intrinsic capacity to incorporate radiotracers for applications as PET nanoprobes. For instance, we have incorporated a radiotracer ( 64 Cu(II)) into NPs for PET imaging through a simple, fast, one-pot, high-yielding radiolabelling strategy (radiochemical yields >96.5%; Fig. 1d ; Supplementary Fig. 19 ). PET imaging showed that 64 Cu NPs started to accumulate at tumour sites 4 h after injection, and reached maximum level at 16 h. After 24 h, the radiolabel was found primarily at the implanted tumours, with very low-background signalling in the rest of the body ( Fig. 6c ). The synergistic combination of PET and MRI is likely to become the next generation of dual-modality scanners to provide accurate diagnoses [31] , [32] . Consequently, there is a great need to develop dual-modality agents that can take advantage of the complementary strengths of PET (high sensitivity and quantifiability) and MR (high soft-tissue resolution) imaging [33] , [34] , [35] . As an exogenous-chelator-free nanoplatform that possesses intrinsic capacity to chelate Gd(III) and radiotracers simultaneously, NPs show significant promise for development as dual-modality nanoprobes for PET-MRI. We have shown that both 64 Cu(II) and Gd(III) could be efficiently incorporated into NPs ( Fig. 1d ; Supplementary Fig. 19 ). Dual-labelled NPs could significantly enhance the MRI contrast and PET signal at the tumour site at 24 h post injection ( Fig. 6d,e ). Interestingly, the heterogeneity of the tumour and the inhomogeneous distribution of NPs in the tumour were noninvasively revealed using PET-MRI ( Fig. 6e ). NPs mediated multimodal therapy in animal models Light-based therapies such as PDT and PTT may offer promising opportunities for cancer treatment [11] , [12] , [36] , [37] , [38] , [39] , [40] , [41] , [42] . There have been studies showing that PTT have synergistic effect with PDT [40] , [43] , [44] . Several inorganic nanoparticle complexes, such as photosensitizer-conjugated gold nanorod [40] , graphene oxide nanoparticles [43] and silica-coated palladium/silver nanoparticles [44] , have been developed for PTT/PDT dual therapy. However, the activation of these nanoparticles required two separate illuminations with multiple-wavelength lasers (for example, 808 and 675 nm) [40] , [43] , [44] . There are also concerns regarding the long-term safety of these inorganic nanoparticles. Here we demonstrated that the biocompatible NPs could be used as a dual-modal nanotransducer that could be activated to release heat and ROS efficiently at tumour site for simultaneous PTT/PDT using a portable, single-wavelength NIR laser. The fluorescence of CNPs stayed quenched in blood after intravenous injection into mice bearing implanted tumour xenograft ( Supplementary Fig. 20 ). Similarly, the ROS production of CNPs in blood was also minimal upon exposure with low-dose light (similar to the sun light at 690 nm received in daily life, 0.1 W cm −2 ; Fig. 7a ). No obvious haemolysis was observed for CNPs in blood after light exposure ( Supplementary Fig. 21 ). The heat generation of CNPs was also negligible after exposure to the same dose of light ( Fig. 7b,c ). To the contrary, NM-POR, the Por-encapsulated conventional micelles, presented five times higher fluorescence in blood of the mice than CNPs and produced significantly higher amount of ROS resulting in severe haemolysis ( Fig. 7a ; Supplementary Figs 20 and 21 ). This is likely because of the less quenching effect of Por molecules when physically encapsulated inside micelles ( Supplementary Fig. 9 ). 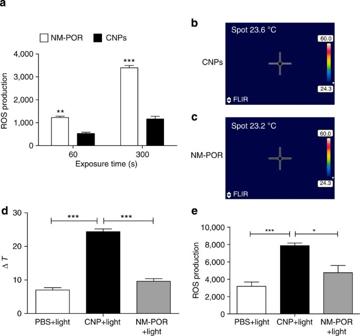Figure 7: ROS production and heat generation in blood and at tumour tissue. (a) ROS production of blood drops drawn from nude mice bearing implanted tumour xenografts 1 min post injection of CNPs and NM-POR (Por dose: 5 mg kg−1) after light exposure and was measured using DCF-DA as ROS indicator (n=3). Light dose: 0.1 W for 60 s and 300 s. The results were expressed as the mean±s.d. **P<0.002, ***P<0.001,t-test. The temperature of blood drops drawn from nude mice bearing implanted tumour xenografts 1 min post injection of (b) CNPs and (c) NM-POR (Por dose: 5 mg kg−1) after light exposure. Light dose: 0.1 W for 300 s. The temperature was monitored by a FLIR thermal camera. (d) The temperature changes (ΔT) at tumours of nude mice bearing implanted SKOV3 tumour xenografts 24 h post injection of PBS, CNPs and NM-POR (Por dose: 5 mg kg−1) after light exposure (n=5). Light dose: 1.25 W cm−2for 120 s. The temperature was monitored using a FLIR thermal camera. The results were expressed as the mean±s.d. ***P<0.001, one-way ANOVA. (e) ROS production at tumours of nude mice bearing implanted tumour xenografts 24 h post injection of PBS, CNPs and NM-POR (Por dose: 5 mg kg−1) after light exposure (n=5). Light dose: 1.25 W cm−2for 120 s. Measured by using DCF-DA as a ROS indicator. The results were expressed as the mean±s.d. *P<0.01, ***P<0.001, one-way ANOVA. Figure 7: ROS production and heat generation in blood and at tumour tissue. ( a ) ROS production of blood drops drawn from nude mice bearing implanted tumour xenografts 1 min post injection of CNPs and NM-POR (Por dose: 5 mg kg −1 ) after light exposure and was measured using DCF-DA as ROS indicator ( n =3). Light dose: 0.1 W for 60 s and 300 s. The results were expressed as the mean±s.d. ** P <0.002, *** P <0.001, t -test. The temperature of blood drops drawn from nude mice bearing implanted tumour xenografts 1 min post injection of ( b ) CNPs and ( c ) NM-POR (Por dose: 5 mg kg −1 ) after light exposure. Light dose: 0.1 W for 300 s. The temperature was monitored by a FLIR thermal camera. ( d ) The temperature changes (Δ T ) at tumours of nude mice bearing implanted SKOV3 tumour xenografts 24 h post injection of PBS, CNPs and NM-POR (Por dose: 5 mg kg −1 ) after light exposure ( n =5). Light dose: 1.25 W cm −2 for 120 s. The temperature was monitored using a FLIR thermal camera. The results were expressed as the mean±s.d. *** P <0.001, one-way ANOVA. ( e ) ROS production at tumours of nude mice bearing implanted tumour xenografts 24 h post injection of PBS, CNPs and NM-POR (Por dose: 5 mg kg −1 ) after light exposure ( n =5). Light dose: 1.25 W cm −2 for 120 s. Measured by using DCF-DA as a ROS indicator. The results were expressed as the mean±s.d. * P <0.01, *** P <0.001, one-way ANOVA. Full size image The tumours were illuminated with therapeutic dose of light (1.25 W cm −2 for 120 s) 24 h after intravenous administration of PBS, CNPs and NM-POR. CNPs were found to elicit 2.5 times temperature increase and generate significantly higher amount of ROS at the tumour site compared with NM-POR ( Fig. 7d,e ; Supplementary Fig. 22 ). Dramatically higher ROS production for CNP-treated group than PBS control group at the illuminated tumour site was further confirmed by using SOSG as an indicator ( Supplementary Fig. 23 ). The simultaneous heat and ROS generation at the tumour site in the CNP-treated group could be attributed to the significant accumulation of CNPs at tumour sites and partial dissociation 24 h after injection ( Fig. 5d ). Upon light irradiation, the intact CNPs are expected to generate heat while the dissociated CNPs could be activated to produce ROS. The above results suggested that architecture-dependent photonic properties of CNPs could be utilized to minimize the unintended toxicity of photosensitizers in blood and to deliver significantly higher amount of heat and ROS to tumour than comparable nanocarriers. We have also demonstrated that the temperature at the tumour site of transgenic mice increased to 57 °C after light irradiation (1.25 W cm −2 for 2 min) 24 h after injection of CNPs ( Fig. 8a,c ). This temperature is sufficient to cause irreversible damage to cancer cells [7] . In contrast, the temperature at the tumour site in the PBS control group only increased to 41°C with identical level of light exposure ( Fig. 8b,c ). The ROS generated by CNPs after irradiation was also significantly higher than the tissue background in the PBS control group, as measured by using DCF-DA ( Fig. 8d ) or SOSG ( Supplementary Fig. 24 ) as indicators. Histopathology revealed large areas of severe tissue damage, such as cellular destruction and apoptosis at 24 h after irradiation ( Fig. 8e ) as evidenced by positive TdT-mediated dUTP nick end labelling results and cleaved caspase3 immunoreactivity ( Supplementary Fig. 25 ). These changes could be attributed to antitumor effects from both heat and ROS production ( Fig. 8a,c,d ). 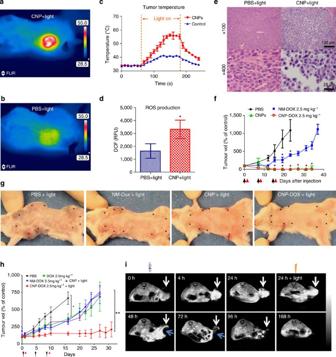Figure 8: Nanoporphyrin-mediated multimodal therapy in animal models and imaging-guided delivery. Representative thermal images of tumours in transgenic mice with mammary cancer (FVB/n Tg(MMTV-PyVmT) after light irradiation at 24 h post injection of (a) CNPs and (b) PBS. (c) Temperature change in tumours in transgenic mice injected with CNPs and PBS before and after irradiation (n=3). The results were expressed as the mean±s.d. (d) ROS production at tumour site in transgenic mice treated with CNPs and PBS (control) for 24 h followed by laser irradiation by using DCF-DA as an indicator (n=3). The results were expressed as the mean±s.d.P<0.025,t-test. (e) Histopathology of tumours from mice injected with PBS or CNPs 24 h after irradiation. The light dose was 1.25 W cm−2for 2 min, while the NPs dose was 25 mg kg−1(equivalent to 5 mg kg−1of Por) fora–e. (f) Tumour volume change of transgenic mice with mammary cancer (n=8) treated with CNPs, CNP-DOX and NM-DOX (standard micelles without porphyrin)21on days 0, 7 and 14 (black arrow) followed by light exposure on the tumours in the mice in all groups at 24 h post injection (red arrow). The results were expressed as the mean±s.d.P<0.01, one-way ANOVA. DOX dose: 2.5 mg kg−1, NP dose: 25 mg kg−1(equivalent to 5 mg kg−1of Por), light dose: 1.25 W cm−2for 2 min. (g) Pictures of transgenic mice on day 34 of the treatment. (*: mammary tumours). (h) Tumour volume change of mice (n=6) bearing SKOV3 ovarian cancer xenograft treated with CNPs and CNP-DOX on days 0, 4 and 8 (black arrow) followed by irradiation on days 1 and 9 (red arrow). PBS and NM-DOX were injected for comparison. DOX dose: 2.5 mg kg−1, NP dose: 25 mg kg−1(equivalent to 5 mg kg−1of Por), light dose: 0.25 W cm−2for 2 min. The results were expressed as the mean±s.d.P<0.01, one-way ANOVA. (i) MRI-guided PTT/PDT: representative MR images of mice injected with Gd-NPs (Gd dose: 0.015 mmol kg−1) before and after laser irradiation. White arrows indicate the tumour sites. Images were collected at 0 (pre-injection), 4, 24, 48, 72, 96 and 168 h post injection. MRI showed large signal voids (blue arrows) at tumour sites 24 h after irradiation (48 h post injection) at a dose of 1.25 W cm−2for 3 min and the tumours were completely ablated at 168 h (7 days) post injection. Figure 8: Nanoporphyrin-mediated multimodal therapy in animal models and imaging-guided delivery. Representative thermal images of tumours in transgenic mice with mammary cancer (FVB/n Tg(MMTV-PyVmT) after light irradiation at 24 h post injection of ( a ) CNPs and ( b ) PBS. ( c ) Temperature change in tumours in transgenic mice injected with CNPs and PBS before and after irradiation ( n =3). The results were expressed as the mean±s.d. ( d ) ROS production at tumour site in transgenic mice treated with CNPs and PBS (control) for 24 h followed by laser irradiation by using DCF-DA as an indicator ( n =3). The results were expressed as the mean±s.d. P <0.025, t -test. ( e ) Histopathology of tumours from mice injected with PBS or CNPs 24 h after irradiation. The light dose was 1.25 W cm −2 for 2 min, while the NPs dose was 25 mg kg −1 (equivalent to 5 mg kg −1 of Por) for a – e . ( f ) Tumour volume change of transgenic mice with mammary cancer ( n =8) treated with CNPs, CNP-DOX and NM-DOX (standard micelles without porphyrin) [21] on days 0, 7 and 14 (black arrow) followed by light exposure on the tumours in the mice in all groups at 24 h post injection (red arrow). The results were expressed as the mean±s.d. P <0.01, one-way ANOVA. DOX dose: 2.5 mg kg −1 , NP dose: 25 mg kg −1 (equivalent to 5 mg kg −1 of Por), light dose: 1.25 W cm −2 for 2 min. ( g ) Pictures of transgenic mice on day 34 of the treatment. (*: mammary tumours). ( h ) Tumour volume change of mice ( n =6) bearing SKOV3 ovarian cancer xenograft treated with CNPs and CNP-DOX on days 0, 4 and 8 (black arrow) followed by irradiation on days 1 and 9 (red arrow). PBS and NM-DOX were injected for comparison. DOX dose: 2.5 mg kg −1 , NP dose: 25 mg kg −1 (equivalent to 5 mg kg −1 of Por), light dose: 0.25 W cm −2 for 2 min. The results were expressed as the mean±s.d. P <0.01, one-way ANOVA. ( i ) MRI-guided PTT/PDT: representative MR images of mice injected with Gd-NPs (Gd dose: 0.015 mmol kg −1 ) before and after laser irradiation. White arrows indicate the tumour sites. Images were collected at 0 (pre-injection), 4, 24, 48, 72, 96 and 168 h post injection. MRI showed large signal voids (blue arrows) at tumour sites 24 h after irradiation (48 h post injection) at a dose of 1.25 W cm −2 for 3 min and the tumours were completely ablated at 168 h (7 days) post injection. Full size image We have shown in Fig. 2 that CNPs could be used as programmable releasing nanocarriers that minimized the drug release in human plasma but could be triggered to release the drug content when exposed to light and intracellular reducing agents. Upon irradiation with NIR light, drug-loaded CNPs are expected be activated to release singlet oxygen, heat and drugs simultaneously at the tumour sites for simultaneous PTT/PDT and chemotherapy. We have performed in vivo therapeutic studies to evaluate the anticancer efficacy of CNPs in transgenic and xenograft mouse models. In the transgenic mammary tumour mouse study, CNP-mediated PTT/PDT could significantly inhibit tumour growth with a light dose of 1.25 W cm −2 for 2 min once per week when compared with the PBS control group and the NM-DOX group. The treated tumours were completely eliminated on day 12 with ulceration ( Fig. 8f ). No palpable tumours were detected even on day 32 ( Fig. 8g ). CNP-DOX-mediated combination therapy of PTT/PDT with DOX showed similar efficacy ( Fig. 8f,g ). In order to effectively compare the efficacy of NP-mediated combination therapy, we will need to use lower dose of NPs and/or lower dose of light. This will be the subject of future work. As expected, in nude mice bearing SKOV3 ovarian cancer xenograft, the NP-mediated phototherapy, free DOX and NM-DOX-treated groups all resulted in slower SKOV3 tumour growth than the PBS control group ( Fig. 8h ). At the same dose of DOX, photosensitizer (porphyrins) and light (0.25 W cm −2 for 2 min), the combination treatment with CNP-DOX showed the best antitumour activity and totally inhibited tumour growth throughout the study ( Fig. 8h ). No significant changes were observed in body weight, complete blood count and serum chemistry after three doses of treatment ( Supplementary Fig. 26 ; Supplementary Table 1 ). Mice were handled without shielding ambient light in the laboratory, but no skin phototoxicity was found. MRI-guided phototherapy As NPs have intrinsic ability to chelate Gd(III), we can conveniently employ MRI to simultaneously monitor in real time the biodistribution of these nanoparticles and the tumour response. As a proof of concept, we used MRI to observe the tumour growth in SKOV3 ovarian cancer mouse models after administration of Gd-NPs with or without illumination ( Fig. 8i ). MR images showed that Gd-NPs had significant accumulation at the tumour site beginning 4 h post injection. For the treatment group, tumours were illuminated at 24 h post injection. MR images at 48 h post injection (24 h after irradiation) showed both shrinkage of the tumour and increase in necrotic volume at the tumour site. MRI showed complete tumour elimination at 7 days post injection. In contrast, MRI showed no difference in tumour size in control mice that were not illuminated. The NP platform reported here possesses several properties that are unique and favourable as theranostic agents: (1) intrinsic ability to chelate imaging agents such as 64 Cu(II) and Gd(III), (2) excellent efficiency for drug-loading, (3) unique architecture-dependent fluorescent, photothermal, photodynamic and magnetic resonance properties, (4) biocompatible, monodisperse and relatively small (20~30 nm) and (5) can be reversibly stabilized via disulphide bonds. We have demonstrated in both ovarian cancer xenograft model and murine transgenic breast cancer model that these novel NPs could be used as: (1) amplifiable nanoprobes to increase the sensitivity of multimodal imaging for tumour detection, (2) nanotransducers that can be activated to generate heat and ROS efficiently at tumour sites for PTT/PDT dual therapy via a single-wavelength light and (3) nanocarriers with programmable releasing property that can minimize the premature drug release in blood and allow efficient release upon light irradiation and/or triggered by the endogenous reducing agent present at the tumour site or in cancer cells [21] . The superior imaging capability of NPs can be further utilized to monitor the real-time in vivo delivery of NPs and for assessing their therapeutic efficacy noninvasively. The results shown above support our concept of using an organic porphyrin nanoconstruct assembled from a single and well-defined polymer unit as a smart and extremely versatile ‘all-in-one’ nanomedicine platform to mediate multimodality imaging (NIRFI, MRI, PET and PET-MRI), as well as PTT, PDT and targeted delivery of drugs or therapeutic radio-metals to tumor. To the best of our knowledge, this is the first report of an organic nanoparticle system that is able to integrate such a broad range of smart and clinically relevant functionalities in a single nano-formulation. The integration of additional functionality into existing nanoparticles will typically increase the cost and the complexity of synthesis, lead to more heterogeneous formulations and affect their in vivo performance [45] . For clinical translation, the cost effectiveness of the nanoplatform must be carefully considered. The present multifunctional NPs were developed based on a single and well-defined building block. The synthesis of porphyrin/CA hybrid telodendrimer is highly reproducible and can be easily scaled-up to kilogram level at relatively low cost. The in vivo performance of NPs remains high in each of its functionality compared with the other nanoparticle systems as discussed below. A variety of fluorescence-labelled nanoparticles [7] , [46] , [47] and quantum dots [8] , [48] have been reported for NIRFI. However, most of these nanoparticles lacked a strategy to minimize the signal in blood and amplify the signal at the tumour site. Porphysome nanovesicles have been found to have structure-dependent fluorescence properties that can be used for low-background NIRFI [7] . However, porphysome nanovesicles are relatively large (~100 nm) resulting in very high uptake in reticuloendothelial system, liver and spleen. NPs are relatively small (20–30 nm); they can be reversibly crosslinked and exhibit unique architecture-dependent fluorescence. Therefore, they are particularly suited as activatable optical nanoprobes to increase the sensitivity of NIRFI for improved cancer detection through background suppression in blood as well as preferential accumulation and signal amplification at the tumour site. This latter property makes NPs particularly useful as probes for image-guided surgery. SPIO-nanoparticles [11] , [12] have been proposed as T 2 -weighted MRI contrast agents but they often suffered from relatively low sensitivity because of their negative contrast [2] , [49] . Nanoparticle-based T 1 -weighted MRI agents usually have excellent contrast enhancement but they often require additional steps for the ligation of chelators [4] , [49] , [50] . The NPs have intrinsic ability to chelate Gd(III) ( Fig. 1d ), preferentially accumulate at the tumour site and possess architecture-dependent magnetic resonance property that allows them to be used as activatable contrast agents for sensitive and tumour-specific MRI. Unlike most other nanoparticles that require added chelation, NPs possess intrinsic ability to directly chelate 64 Cu(II) that allows not only their biodistribution but also pharmacokinetics to be noninvasively tracked in vivo by PET. Furthermore, NPs can chelate Gd(III) and radiotracers simultaneously, making it a promising dual-modality nanoimaging agent for combined PET-MRI. There have been studies showing that PTT has synergistic effect with PDT and could enhance the outcome of PDT and chemotherapy by increasing local permeability of the sensitizer and drugs [40] , [43] , [44] . Here we demonstrated in vivo that the ‘soft’ organic NPs could be employed for simultaneous PTT/PDT using a portable, single-wavelength NIR laser. The architecture-dependent photonic properties of NPs could be utilized to minimize the unintended toxicity of photosensitizers in blood, and deliver significantly higher amount of ROS and heat to tumour than comparable nanocarriers. Although NPs can in principle reach tumour sites throughout the body, PTT and PDT, however, are limited by the region of the body accessible to light irradiation and the depth of NIR laser penetration into tissues. The improvements in light delivery methods [51] and targeting property of NPs via targeting moieties for specific type of tumours [52] will undoubtedly further increase the therapeutic efficacy and accelerate the translation of such NPs to the clinic. NPs can be used as a non-toxic nanoplatform for hydrophobic anticancer drug formulation, yielding relatively small and monodisperse nanotherapeutics with high drug-loading efficiency. To minimize premature drug release in the circulation, NPs can be crosslinked by disulphide bonds. Such CNPs can be triggered to release the drug content by light exposure and intracellular reducing agents. The current configuration of our NPs is designed to carry hydrophobic drugs. Further modifications of the NPs, however, will be needed if we want to deliver hydrophilic payloads such as DNA, RNA, proteins and enzymes. In addition to achieving and validating the nanoscale integration of imaging and therapeutic functions, it is important to demonstrate the benefits and synergy of such a combined approach. We have demonstrated that NPs could be activated to release singlet oxygen, heat and drugs simultaneously at the tumour sites for simultaneous PTT/PDT and chemotherapy upon illumination. This synergistic approach will make PTT/PDT much more effective. For tumours that are beyond the reach of the light, antitumor effects can still be achieved with a chemotherapeutic agent such as PTX and DOX encapsulated inside the NPs. We have also shown that the unique MRI capabilities of NPs could be utilized to conveniently monitor the biodistribution of NPs as well as their therapeutic efficacy, including the tumour size and necrosis inside the tumour after PTT/PDT. This integrated nanomedicine platform shows great promise as a highly versatile multimodal theranostic agent against cancers. Synthesis of telodendrimers The representative porphyrin/CA hybrid telodendrimer (PEG 5k -Por 4 -CA 4 , Fig. 1a ; Supplementary Fig. 1 ) was synthesized via solution-phase condensation reactions from MeO-PEG-NH 2 utilizing stepwise peptide chemistry according to our published methods [16] . Briefly, (Fmoc)Lys(Fmoc)-OH (3 eq.) was coupled on the N terminus of PEG using DIC and HOBt as coupling reagents until a negative Kaiser test result was obtained, thereby indicating completion of the coupling reaction. PEGylated molecules were precipitated by adding cold ether and then washed with cold ether twice. Fmoc groups were removed by the treatment with 20% (v/v) 4-methylpiperidine in dimethylformamide (DMF), and the PEGylated molecules were precipitated and washed three times by cold ether. White powder precipitate was dried under vacuum and one coupling of (Fmoc)Lys(Fmoc)-OH and one coupling of (Fmoc)lys(Boc)-OH were carried out, respectively, to generate a third generation of dendritic polylysine terminated with four Boc and Fmoc groups on one end of PEG. CA NHS ester [16] and pyropheophorbide-a were coupled to the terminal end of dendritic polylysine after the removal of Fmoc with 20% (v/v) 4-methylpiperidine and the removal of Boc groups with 50% (v/v) trifluoroacetic acid in dichloromethane, respectively. The telodendrimer solution was filtered and then dialysed against 4 l water in a dialysis tube with MWCO of 3.5 KDa; reservoir water was refreshed completely four times in 24 h. Finally, the telodendrimer was lyophilized. The molecular weight of PEG 5k -Por 4 -CA 4 was collected on ABI 4700 MALDI-TOF/TOF mass spectrometer (linear mode) using R-cyano-4-hydroxycinnamic acid as a matrix. The monodispersed mass traces were detected for the telodendrimers, and the molecular weight of the telodendrimer from MALDI-TOF MS ( Supplementary Fig. 2 ) was almost identical to the theoretical value. 1 H NMR spectra of the telodendrimers were recorded on an Avance 500 Nuclear Magnetic Resonance Spectrometer (Bruker) using DMSO-d6 and D2O as solvents. The concentration of the telodendrimers was kept at 5 × 10 −4 M for NMR measurements ( Supplementary Fig. 3 ). The thiolated pyropheophorbide-a telodendrimer (named as PEG 5k -Cys 4 -Por 4 -CA 4 , Fig. 2a ; Supplementary Fig. 10 ) was synthesized by replacing four of the eight CAs of our previously reported thiolated telodendrimer (PEG 5k -Cys 4 -L 8 -CA 8 ) using the same strategy [16] , [21] . The typical procedure for synthesis of PEG 5k -Cys 4 -Por 4 -CA 4 was as follows: (Fmoc)Lys(Fmoc)-OH (3 eq.) was coupled on the N terminus of PEG using DIC and HOBt as coupling reagents until a negative Kaiser test result was obtained, thereby indicating completion of the coupling reaction. PEGylated molecules were precipitated by adding cold ether and then washed with cold ether twice. Fmoc groups were removed by the treatment with 20%(v/v) 4-methylpiperidine in DMF, and the PEGylated molecules were precipitated and washed three times by cold ether. White powder precipitate was dried under vacuum and one coupling of (Fmoc)Lys(Fmoc)-OH and one coupling of (Dde)lys(Fmoc)-OH were carried out, respectively, to generate a third generation of dendritic polylysine terminated with four Dde and Fmoc groups on one end of PEG. Then the Fmoc groups were removed. (Fmoc)Cys(Trt)-OH, (Fmoc)Ebes-OH and CA NHS ester (12 eq.) were coupled step by step to the terminal end of dendritic polylysine. After the removal of Dde protecting group by 2%(v/v) hydrazine in DMF, (Fmoc)Ebes-OH and pyropheophorbide-a (12 eq.) were coupled subsequently to the leftover amino groups on the terminal end of dendritic polylysine. The Trt groups on cysteines were removed by trifluoroacetic acid/H2O/ethanedithiol/triethylsilane (94:2.5:2.5:1, v/v) resulting in PEG 5k -Cys 4 -Por 4 -CA 4 -thiolated telodendrimer ( Fig. 2a ; Supplementary Fig. 10 ). The thiolated telodendrimer was recovered from the mixture by three cycles of dissolution/reprecipitation with DMF and ether, respectively. Finally, the thiolated telodendrimer was dissolved in acetonitrile/water and lyophilized. The molecular weight of PEG 5k -Cys 4 -Por 4 -CA 4 was collected on ABI 4700 MALDI-TOF/TOF mass spectrometer (linear mode) using R-cyano-4-hydroxycinnamic acid as a matrix. The monodispersed mass traces were detected for the starting PEG and the telodendrimers, and the molecular weights of the telodendrimers from MALDI-TOF MS ( Supplementary Fig. 11 ) were almost identical to the theoretical value. Preparation of NPs In all, 20 mg thiol-free porphyrin–telodendrimer was dissolved in 1 ml PBS followed by sonication for 10 min to form NPs. In order to make CNP, 20 mg total amount of PEG 5k -Cys 4 -Por 4 -CA 4 was dissolved in 1 ml PBS to form micelles and then sonicated for 10 min. The thiol groups on the telodendrimer were oxidized to form disulphide linkages by air [21] . Generation of metallic NPs To generate telodendrimers with a chelated metal, excess free metal ions were incubated with telodendrimers in methanol/chloroform for 1–5 h under nitrogen according to previously reported methods [7] , [53] . Free metal was removed by column filtration with a molecular weight cutoff of 3,500. The metal–telodendrimer was then aliquoted and dried. Metallic NPs were generated by dissolving the metal–telodendrimer in PBS with sonication. Preparation of drug-loaded NPs Hydrophobic drugs, such as DOX, were loaded into NPs by the solvent evaporation method [21] , [24] . Before the encapsulation of DOX into NPs, DOX˙HCl was stirred with 3 molar equivalent of triethylamine in chloroform (CHCl 3 )/methanol (MeOH; 1:1, v/v) overnight to remove HCl from DOX˙HCl. In all, 20 mg porphyrin–telodendrimer along with different amounts of neutralized DOX were first dissolved in CHCl 3 /MeOH, mixed and evaporated on rotavapor to obtain a homogeneous dry polymer film. The film was reconstituted in 1 ml PBS, followed by sonication for 30 min, allowing the sample film to disperse into NP solution. Finally, the NP solution was filtered with a 0.22-μm filter to sterilize the sample. To determine the amount of drugs, drug-loaded NPs were diluted with DMSO (NP solution/DMSO: 1:9, v/v) to dissociate nanoparticles. The drug-loading was analysed on an HPLC system (Waters), wherein calibration curve was obtained using a series of drug/DMSO standard solutions with different concentrations. The drug-loaded CNPs were prepared via the same method followed by the oxidation of the thiols to form intramicellar disulphide bonds [21] . Characterizations of NPs The size and size distribution of NPs were measured by DLS instruments (Microtrac). The concentrations were kept at 1.0 mg ml −1 for DLS measurements. All measurements were performed at 25 °C, and data were analysed with the Microtrac FLEX Software 10.5.3. The morphology of NPs was observed on a Philips CM-120 TEM. Briefly, the aqueous nanoparticle solution (1.0 mg ml −1 ) was deposited on copper grids, with or without staining by phosphotungstic acid for 2 s and measured at room temperature. The size of the particles was analysed with the TEM software (DigitalMicrograph, Gatan Inc). The absorbance and the fluorescence signals of NPs were measured on a fluorescence spectrometry (SpectraMax M2, Molecular Devices, Sunnyvale, CA, USA). The near-infrared fluorescence of NP solutions (10 μl) was scanned using a Kodak multimodal imaging system IS2000MM. The thermo property of NP solutions (10 μl) was studies using a FLIR thermal camera. The ROS production of NPs was studied using SOSG or 2′,7′-Dichlorofluorescin diacetate (DCF-DA) as an indicator and compared with PBS. Briefly, SOSG and/or DCF-DA working solution was mixed with different concentrations of NPs/CNPs with and without SDS (2.5 mg ml −1 ) and GSH (10 mM) in 96-well plate. After 20 s of NIF light exposure, green fluorescence was monitored by micro-plate reader (SpectraMax M2, Molecular Devices). Stability of NPs in SDS and human plasma The stability study was performed to monitor the change in fluorescence and particle size of NPs and CNPs in the presence of SDS, which was reported to be able to efficiently break down polymeric micelles [54] . An SDS solution (7.5 mg ml −1 ) was added to aqueous solutions of NPs (1.5 mg ml −1 ). The final SDS concentration was 2.5 mg ml −1 and the micelle concentration was kept at 1.0 mg ml −1 . The fluorescence signal of the solutions was measured on micro-plate reader (SpectraMax M2). The size and size distribution of the NP solutions were monitored at predetermined time intervals by DLS. The stability of the micelles was also evaluated in the presence of GSH (20 mM) together with SDS. The stability of DOX-loaded NPs was further studied in 50% (v/v) plasma from healthy human volunteers. The mixture was incubated at physiological body temperature (37 °C) followed by size measurements at predetermined time intervals up to 48 h. DOX release in human plasma CNP-DOX solutions were prepared to determine the in vitro drug release profile in plasma. The initial DOX concentration was 1.0 mg ml −1 while the CNP concentration was 10 mg ml −1 . CNP alone and our reported standard micelles (without porphyrins) with DOX at the same drug content were also prepared for comparison. When DOX was encapsulated in the core of CNPs, the proximity between DOX and Por was within the FRET range allowing efficient energy transfer from DOX to Por molecules upon excitation of DOX at 480 nm ( Fig. 2e,f ). Upon excitation at 480 nm, the signal of CNPs alone was much smaller in comparison with the corresponding FRET signal. Therefore, by monitoring the dynamic change of FRET ratio, we were able to monitor the release of DOX from CNPs in real time. Aliquots of these nanoparticle solutions were diluted nine times by human plasma and incubated in an incubator at 37 °C with a stirring speed of 100 r.p.m. The fluorescence spectra of these nanoparticle solutions were measured using NanoDrop spectrophotometer (Thermo Scientific) at predetermined time points. The in vitro DOX release profiles from CNPs were further measured by the dialysis method [21] . In some experiments, aliquots of DOX-loaded NP solution were pretreated with light or GSH (10 mM) or no treatment and then dialysed against diluted human plasma. The concentrations of DOX at different time points were measured using a Molecular Devices SpectraMax M2 at excitation 470 nm/emission 590 nm. Data were reported as the average percentage of DOX accumulative release for each triplicate sample. In vitro cell uptake and cytotoxicity To study the intracellular delivery of DOX-loaded NPs, SKOV3 ovarian cancer cells were seeded on eight-well chamber slides and treated with CNP-DOX (0.1 mg ml −1 DOX) in solution containing Hoechst 33342 for 2 h. Cell imaging was acquired using Deltavision deconvolution microscope. SKOV3 ovarian cancer cell lines were used to evaluate the photosensitizing function of CNPs. We first treated the cancer cells with various concentrations of CNPs or 5-ALA, the traditional photodynamic diagnosis/therapy agent, for 24 h. After thorough washing, the cells were exposed to NIF light as indicated. Cell viability was determined using WST-8 proliferation kit 24 h after illumination. In another experiment, CNPs or DOX-loaded CNPs, free DOX and DOX-loaded crosslinked micelles (without porphyrins) [21] were used to treat the cancer cells for 24 h. After three times of wash, cells were illuminated with light for 1 min. Cell viability was determined by WST-8 after 24 h of incubation. ROS production and cell death mechanisms We first treated SKOV3 cells with or without 10 μg ml −1 of CNPs for 24 h followed by 30 min loading with DCF-DA in 96-well plate to monitor the ROS production. Cells were washed three times with PBS and replaced with fresh medium. A portion of the well was illuminated with NIR light and cell imaging was acquired under fluorescence microscope using the Metamorph programme. Next, to evaluate the loss of mitochondrial membrane potential (Δ Ψ m) after pretreated SKOV3 cells with NPs, we loaded cells with 40 nM of DiOC 6 (3) for 20 min and a portion of the well was illuminated with NIR light. Twenty-four hours later, cells were labelled with propidium iodide (dead cells) and Hoechst 33342 (nucleus), and imaging was acquired using fluorescence microscope. Last, to investigate the cellular responses to CNPs and phototherapy, we evaluated the caspase 3/7 activity, which served as marker for a part of apoptosis pathway activation. SKOV3 cells were treated with or without 10 μg ml −1 CNPs for 24 h. After wash, cells were exposed without light or light for 0.5, 1 and 2 min. After 24 h of incubation, caspase3/7 activity was measured by adding another 50 μl of working solution for another 45 min. The plate was read by microplate reader (SpectraMax M2). Last, for morphology study, SKOV3 cells were cultured on eight-well chamber slides and treated with or without CNPs for 24 h. Two hours after treatment with light, the slide was stained with Hema3 and observed under light microscope. Animal models Female athymic nude mice (Nu/Nu strain), 6–8 weeks of age, were purchased from Harlan (Livermore, CA, USA). All animal experiments were performed in compliance with the institutional guidelines and according to protocol No. 07-13119 and No. 09-15584 approved by the Animal Use and Care Administrative Advisory Committee at the University of California, Davis. The subcutaneous xenograft model of ovarian cancer and lung cancer was established by injecting 2 × 10 6 SKOV3 ovarian cancer cells or A549 lung cancer cells in a 100 μl of mixture of PBS and Matrigel (1:1 v/v) subcutaneously into the right flank of female nude mice, respectively. Female transgenic mice with mammary cancer (FVB/n Tg(MMTV-PyVmT)) were ordered from Jackson Laboratory. Those mice were known to spontaneously developed mammary cancers at the ages of 4–40 weeks. In vivo blood elimination kinetics The jugular vein of male Sprague–Dawley rats was cannulated and a catheter was implanted for intravenous injection and blood collection (Harland, Indianapolis, IN, USA). NPs and CNPs at identical porphyrin concentration were injected through the catheter at a dose of 5 mg kg −1 body weight ( n =3 for each group). Whole blood samples (~100 μl) were collected via jugular vein catheter before dosing and at predetermined time points post injection and used to detect porphyrin concentration by the measurement of absorbance at 680 nm on micro-plate reader (SpectraMax M2). The values were plotted versus time after the subtraction of blood background. NIRF imaging After transgenic mice (10–12 weeks) and nude mice developed established tumours (6–10 mm in diameter), they were subjected to in vivo NIRF imaging by injecting 100 μl of NPs via tail vein. At different time points post injection of NPs, mice were scanned using a Kodak multimodal imaging system IS2000MM with an excitation bandpass filter at 625/20 nm and an emission at 700/35 nm under anaesthesia. After in vivo imaging, animals were killed. Tumours and major organs were excised and imaged with the Kodak imaging station. To monitor the kinetics of biodistribution at the tissue level, SKOV3 tumour-bearing mice were given 100 μl of CNPs via tail vein and killed at 1, 24 or 48 h. Right before euthanasia, Dextran-FITC solution was injected intravenously to locate blood vessel. Tumours were harvested and fixed in the cold formalin on ice. A fresh cross-section was made for LSI laser scanning confocal microscope imaging. In additional, lungs with metastatic lesions were also collected from older transgenic mice (20–24 weeks) and fixed in cold formalin for 1 h. The lung surface was imaged using LSI laser scanning confocal microscopy. After imaging, lungs were subjected to histopathological evaluation. In some cases, the blood of the mice were drawn and measured at predetermined time points. Radiolabelling 64 CuCl 2 in 0.1 M HCl (Washington University, MO, USA) was buffered with 1.0 M ammonium acetate to pH 7. PEG 5k -Por 4 -CA 4 telodendrimer was dissolved in methanol before adding a small volume of buffered 64 CuCl 2 . The radiolabelling solution was incubated for 30 min at room temperature. The methanol was evaporated and the film of telodendrimers was rehydrated with PBS to generate 64 Cu-labelled NPs. Free 64 Cu was removed by centrifuged filtration using 3,500 kDa cutoff Amicon centrifugal filter units (Millipore, Billerica, MA, USA), or alternatively, Micro Bio-Spin 6 columns (Bio-Rad, Hercules, CA, USA). Radiochemical purity and yield were assessed using instant thin-layer chromatography. To prepare dual-labelled Gd/ 64 Cu NPs, pre-prepared Gd-telodendrimer was added to 64 Cu-PEG 5k -Por 4 -CA 4 telodendrimer radiolabelling solution in methanol, followed by drying, reconstitution in PBS and purification. MRI and PET imaging The in vitro MRI signal enhancement of Gd-NPs in the absence and in the presence of SDS was obtained using a Bruker Biospec 7T MRI scanner using T1-weighted Fast Low Angle SHot (FLASH) sequence (echo time (TE)/repetition time (TR)=4/200 ms) using a 128 × 128 matrix size. Nude mice bearing SKOV3 ovarian cancer xenograft, nude mice bearing A549 lung cancer xenografts and transgenic mice with mammary cancer (FVB/n Tg(MMTV-PyVmT) were imaged on a Bruker Biospec 7T MRI scanner. Spin echo images were acquired to determine solid tumour location and volume. To assess the kinetics of the Gd-NPs in the body and tumour as well as the nanoparticle-enhanced MRI signal intensity, a dynamic T1-weighted FLASH sequence was used to acquire images just before injection and at predetermined time points post injection of Gd-NPs (Gd dose: Gd dose: 0.015–0.02 mmol kg −1 ) (TE/TR=4/200 ms) using a 128 × 128 matrix size. MRI was also used to monitor the tumour growth in nude mice bearing SKOV3 ovarian cancer xenografts before and after PTT/PDT using the same parameters. PET was performed on nude mice bearing SKOV3 ovarian cancer xenografts post injection of 64 Cu-labelled NPs (described in Supplementary Methods ; 150–200 μl, 64 Cu dose: 0.6–0.8 mCi) on a small-animal microPET system (Siemens Inveon D-PET). PET-MRI was performed on a small-animal microPET system (Siemens Inveon D-PET) and a Bruker Biospec 7T MRI scanner. Nude mice bearing A549 lung cancer xenografts were placed on a movable bed that fits into both scanners in order to facilitate co-registration of the PET and MR images. After tail vein injection of 64 Cu and Gd dual-labelled NPs (described in Supplementary Methods ; 150–200 μl, 64 Cu dose: 0.6–0.8 mCi, Gd dose: 0.015–0.02 mmol kg −1 ), the mice were imaged under anaesthesia (2% isoflurane in oxygen at 2 l min −1 ) at 4 or 24 h post injection. Amide software was used to co-register the PET and MR images. In vivo therapeutic studies Transgenic mice with mammary cancer (FVB/n Tg(MMTV-PyVmT) and nude mice bearing SKOV3 ovarian cancer xenograft were used for the in vivo therapeutic studies. When tumour volumes reached 4–5 mm in transgenic mice, CNPs with and without 2.5 mg kg −1 DOX were injected via tail vein once per week for three doses. After 24 h, tumours were illuminated with a diode laser system (Applied Optronics, Newport, CT, USA) at 690 nm under general anaesthesia. The light dose was 1.25 W cm −2 for 2 min through an optical fibre producing a 0.8 cm 2 beam spot to cover the whole tumour. Tumour surface temperatures were monitored with a thermal camera (FLIR). The temperature readings in the central point of the illumination area were recorded continuously. Intratumoral ROS production after irradiation was measured using DCF-DA and/or SOSG as indicators. In some cases, the blood of the mice was drawn and the ROS and heat production in blood after irradiation were measured at predetermined time points. The haemolysis was also followed. Tumour volume was measured twice a week and mice were killed once the tumour size reached 1,000 mm 3 . Tumours were harvested for histopathological evaluation 24 h post irradiation. The SKOV3 ovarian cancer xenograft model was established by injecting one million cells subcutaneously at lower flank area. After the tumours reached 150–200 mm 3 , mice received PBS, 2.5 mg kg −1 DOX and CNPs with and without 2.5 mg kg −1 DOX every 3 days for three doses. Laser light (0.2 W cm −2 ) was given for 2 min after dose 1 and 3. Tumour sizes and body weight were measured twice a week, while mice were monitored daily for potential signs of toxicity. Two days after the last dose, CBC and serum chemistry were performed. One mouse from each group was also killed and the major organs were harvested for histopathology evaluation. Statistical analysis Statistical analysis was performed by Student’s t -test for two groups, and one-way analysis of variance for multiple groups. All results were expressed as the mean±s.d. unless otherwise noted. A value of P <0.05 was considered statistically significant. How to cite this article: Li, Y. et al. A smart and versatile theranostic nanomedicine platform based on nanoporphyrin. Nat. Commun. 5:4712 doi: 10.1038/ncomms5712 (2014).